Widom line and dynamical crossovers as routes to understand supercritical water Supercritical water is fundamental in many fields of applications and a precise characterization of the supercritical state is of uttermost importance for this liquid. In a fluid, when moving from the critical point into the single-phase region, the thermodynamic response functions show maxima reminiscent of the critical divergence. Here we study the thermodynamic properties of water in the supercritical region by analysing both available experimental data and our computer simulation results. We find that the lines connecting the maxima of the response functions converge on approaching the critical point in a single line, the Widom line. We further show that the Widom line coincides with a crossover from a liquid-like to a gas-like behaviour clearly visible in the transport properties. These thermodynamic and dynamic features show that the supercritical state in water is far more complex than what was so far believed, indicating a new perspective in the characterization of the thermodynamics of this state. The coexistence between the gas and the liquid phases of a system terminates in a critical point, determined by the critical temperature T C and pressure P C . Beyond this point, for temperatures T > T C and pressures P > P C the two phases merge in a single supercritical fluid phase where gas and liquid are considered indistinguishable. Supercritical fluids are present in nature, for instance, in submarine volcanoes or in atmospheres of giant planets. Among the different fluids, the study of thermodynamic, structural and dynamical properties of water in the supercritical phase plays the most crucial role in chemical engineering, in carbon capture and storage, in pharmaceutics, in waste disposal and in several other areas of applications [1] , [2] such as gasification of biomasses [3] , [4] . The studies of the supercritical region have been so far limited by technical difficulties in experiments, but the investigation of supercritical water is of great interest for understanding its physical properties [5] , [6] . The range of the supercritical region extends for T > T C and P > P C , where T C =647.096 K and P C =220.640 bar, and it is upper bounded by the melting line between supercritical water and high pressure ice of type VII [7] , [8] . It is well known that water shows many peculiar features in all its phases and a great effort has been devoted to the study of this system in the thermodynamic space from ambient conditions down to crystallization/vitrification and up in temperature to the liquid–gas transition [9] , [10] . The challenge in this field is to find unifying concepts that can be used to describe the behaviour of water in the different phases, including the supercritical phase. In this context is the concept of Widom line (WL) [5] is particularly useful. The concept of WL came to the fore in the last few years where it was extensively considered in supercooled water in connection with the possible existence of a liquid–liquid transition terminating in a second critical point [11] , [12] , [13] , [14] , [15] , [16] , [17] , [18] , [19] , [20] , [21] , [22] . In a fluid, when moving from the critical point to the single-phase region, it is expected that the correlation length keeps a maximum reminiscent of the critical divergence. On approaching the critical point from this region, quantities such as the specific heat and the isothermal compressibility show maxima that are expected to merge on a pseudo-critical single line terminating at the critical point. The maxima of those response functions collapse on the same line on approaching the critical point, as they become proportional to power laws of the correlation length. This line, called the WL, has been introduced to define this locus of maxima extending from the critical point into the single-phase region [5] . Entering into the single-phase region, the maxima are smeared out progressively and their values decrease. The WL of supercritical noble gases, Lennard–Jones and van der Waals fluids was recently studied by experiments and simulations [23] , [24] , [25] , [26] , [27] . In particular, a recent experimental work has paved the way to a more profound knowledge of hot dense fluids by detecting a crossover in sound velocity of supercritical fluids of noble gases connected to the WL [26] . Moreover, in the case of water the existence and range of persistence of the WL in the supercritical state can be of great interest, as it can indicate the limiting pressure and temperature values for which the dissolving ability of supercritical water and its other technological important features can be exploited. In this work, we show that the WL does exist in supercritical water and we identify its exact location in the phase diagram. Besides, we demonstrate that there is also a dynamic crossover on crossing the WL that witnesses the strict connection between dynamics and thermodynamics in supercritical water similar to that found for supercritical noble gases [26] . We also determine the range of temperatures above the liquid–gas critical point (LGCP), for which all thermodynamic and dynamic quantities converge on a single WL. Thermodynamic properties in the supercritical region To identify the WL, we did analyse available data obtained from IAPWS-95/IAPS-85 equation of states (EoS), based on experimental data (see Methods), and we performed molecular dynamics simulations with the TIP4P/2005 potential [28] . We chose to use the TIP4P/2005, because among all atom models of that kind it gives the critical temperature and density closest to the experimental findings [29] . The values of the critical parameters from experiments are T C =647.096 K, P C =220.640 bar and ρ C =0.322 g cm −3 and TIP4P/2005 gives T C =640 K, P C =146 bar and ρ C =0.31 g cm −3 . In Fig. 1a we present the experimental isobars of water in the supercritical region, while in Fig. 1b we show the isobars calculated for the TIP4P/2005 potential. In both cases, the isobars are shown for temperatures between T =600 K and T =800 K, and for pressures approximately at the same distance from the respective critical values: P n =220+25 n bar for experimental water and P n =150+25 n bar for TIP4P/2005 water, with n =1,...,10. As such, these isobars span a zone of the P − T diagram that goes from the liquid region to the supercritical region. Furthermore, the selected isobars never cross the liquid–gas coexistence line and therefore discontinuous jumps are not to be expected. Looking at Fig. 1a,b , we immediately note that the TIP4P/2005 model reproduces extremely well the envelope of the experimental isobars, albeit with the shift in pressure. 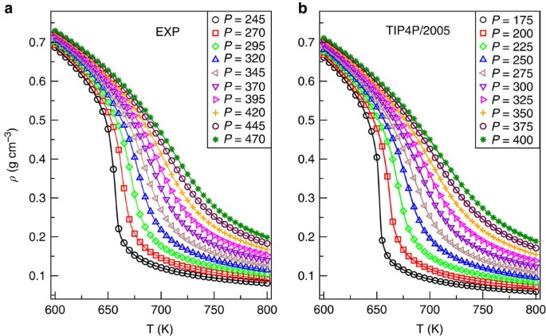Figure 1: Supercritical isobars from experiments and TIP4P/2005. (a) Isobars for experimental water between 600 and 800 K, and for pressuresPn=220+25nbar (n=1,...,10). (b) Isobars for the TIP4P/2005 between 600 and 800 K, and for pressuresPn=150+25nbar (n=1,...,10). In both panels, each colour corresponds to the samenin the formulas for the pressure, and as such it indicates the same distance from the respective critical point. The lines are obtained by spline interpolations. Figure 1: Supercritical isobars from experiments and TIP4P/2005. ( a ) Isobars for experimental water between 600 and 800 K, and for pressures P n =220+25 n bar ( n =1,...,10). ( b ) Isobars for the TIP4P/2005 between 600 and 800 K, and for pressures P n =150+25 n bar ( n =1,...,10). In both panels, each colour corresponds to the same n in the formulas for the pressure, and as such it indicates the same distance from the respective critical point. The lines are obtained by spline interpolations. Full size image To find the location of the WL, we determined for both experimental and simulation data the maxima of three thermodynamic response functions. The constant pressure-specific heat C P defined as where H is the enthalpy. The expansion coefficient α P defined as and the isothermal compressibility K T defined as The behaviour of C P is shown in the inset of Fig. 2 as extracted from experimental data for pressures above the LGCP. In spite of the fact that we are in the one-phase region, the specific heat peak is very well defined also for pressure that are quite far from the LGCP. The same persistence of defined maxima well above the LGCP is found also in simulations and for α P and K T (not shown). 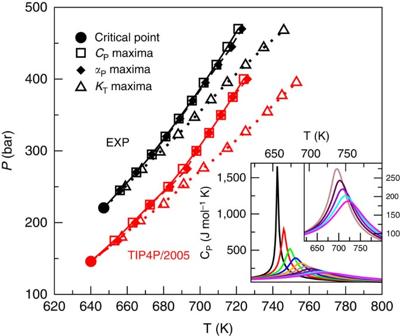Figure 2: The Widom lines from experiments and TIP4P/2005. Main Frame: critical points (circle) andP−Tlocation of the maxima ofCP(squares),αP(diamonds) andKT(triangles) as reproduced by experimental data (black) and by the molecular dynamics simulations performed using the TIP4P/2005 model (red). The definitions of the functions are provided in the text. All maxima were calculated along isobars. Lines are guides for the eye. Values for the critical point are respectively: from experimentsTC=647.096 K,PC=220.640 bar andρC=0.322 g cm−3and from computer simulationsTC=640 K,PC=146 bar andρC=0.31 g cm−3. Inset: experimental isobaric specific heatCPas a function of temperature for pressuresPn=220+25nbar (n=1,...,10) above the critical pressure. The sub-inset shows a magnification for pressuresP≥370 bar. The lines are obtained directly from the linear interpolation of the data with ΔT=1 K. Figure 2: The Widom lines from experiments and TIP4P/2005. Main Frame: critical points (circle) and P − T location of the maxima of C P (squares), α P (diamonds) and K T (triangles) as reproduced by experimental data (black) and by the molecular dynamics simulations performed using the TIP4P/2005 model (red). The definitions of the functions are provided in the text. All maxima were calculated along isobars. Lines are guides for the eye. Values for the critical point are respectively: from experiments T C =647.096 K, P C =220.640 bar and ρ C =0.322 g cm −3 and from computer simulations T C =640 K, P C =146 bar and ρ C =0.31 g cm −3 . Inset: experimental isobaric specific heat C P as a function of temperature for pressures P n =220+25 n bar ( n =1,...,10) above the critical pressure. The sub-inset shows a magnification for pressures P ≥370 bar. The lines are obtained directly from the linear interpolation of the data with Δ T =1 K. Full size image The maxima of C P , α P and K T are reported for both experiments and simulations in the main frame of Fig. 2 . As the most important finding we note that both for the experimental data and for the simulation data, the C P , α P and K T lines perfectly coincide in a certain range above the LGCP as expected from the theoretical interpretation of the WL. We do see that this range extends circa 30 K and 90 bar above the LGCP for both experiments and simulations. Further away from the LGCP C P and α P lines keep on coinciding, while K T deviates. Apart from the small shift to lower pressures of the LGCP position, the agreement between the TIP4P/2005 and experiments for C P , α P and K T lines is remarkable. Transport properties in the supercritical region We consider now the transport properties in the supercritical region. The more extended experimental results for water in the supercritical range have been found for the viscosity η , which is reported in Fig. 3a . In the plot, we also marked the values of η corresponding to the P- and T -values of the experimental WL defined in the previous section. When the curves defining the WL start to separate, we marked the η corresponding to the maxima of the isobaric specific heat. 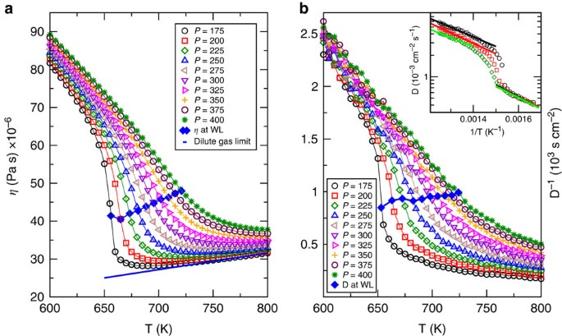Figure 3: Viscosity from experiments and diffusion coefficient from simulations. (a) Viscosity from experiments for different pressures (in bar). The curves are interpolations of the data and the diamonds are the values ofηinterpolated at the points of experimental WL and/orCpmaxima. The bold line is the viscosity in the dilute gas limit31. (b) Diffusion coefficients as obtained from simulations with the TIP4P/2005 potential along the isobars (the lines are guides for the eyes). The diamonds are the values ofDinterpolated at the points of WL and/orCpmaxima given by the model and reported inFig. 2. In the inset, the coefficientDfor the lowest pressures are reported as function of 1/T; the bold lines are the fitting with the equation (4); the activation energies are: for highT,EA=25.7 kJ mol−1forP=175 bar,EA=28.2 kJ mol−1forP=200 bar,EA=23.8 kJ mol−1forP=225 bar; for lowT,EA=31.5 kJ mol−1forP=175 bar,EA=28.7 kJ mol−1forP=200 bar,EA=30.8 kJ mol−1forP=225 bar. Figure 3: Viscosity from experiments and diffusion coefficient from simulations. ( a ) Viscosity from experiments for different pressures (in bar). The curves are interpolations of the data and the diamonds are the values of η interpolated at the points of experimental WL and/or C p maxima. The bold line is the viscosity in the dilute gas limit [31] . ( b ) Diffusion coefficients as obtained from simulations with the TIP4P/2005 potential along the isobars (the lines are guides for the eyes). The diamonds are the values of D interpolated at the points of WL and/or C p maxima given by the model and reported in Fig. 2 . In the inset, the coefficient D for the lowest pressures are reported as function of 1/ T ; the bold lines are the fitting with the equation (4); the activation energies are: for high T , E A =25.7 kJ mol −1 for P =175 bar, E A =28.2 kJ mol −1 for P =200 bar, E A =23.8 kJ mol −1 for P =225 bar; for low T , E A =31.5 kJ mol −1 for P =175 bar, E A =28.7 kJ mol −1 for P =200 bar, E A =30.8 kJ mol −1 for P =225 bar. Full size image It is known that η at the critical point has a power law divergence with a small exponent [30] , [31] . The curves of η in the supercritical zone on approaching the critical pressure show a reminiscence of the critical behaviour with an almost vertical change with temperature. The WL signs a change of behaviour of the viscosity from liquid like to gas like. In fact, in the liquid-like portion, all curves show a strong decrease of viscosity with temperature. In the gas-like portion, the change of slopes is more mild. We note that at low densities the viscosity increases with temperature as predicted by theoretical approaches [32] . The increase is well fitted at low pressures by the formula for the viscosity in the dilute gas limit [31] as shown in Fig. 3a . At increasing pressure, the dense water gas far from the dilute limit shows a change of trend and the viscosity mildly decreases with temperature. The diffusion coefficient D of supercritical water calculated with the molecular dynamics simulation of TIP4P/2005 is shown in Fig. 3b . Moreover, in the plot of the diffusion coefficient we did mark the values of D corresponding to the P- and T -values of the TIP4P/20005 WL defined in the previous section. When the curves defining the WL start to separate, we marked the D corresponding to the maxima of the isobaric specific heat. In approaching the critical pressure, the variations of the diffusion coefficient become more drastic. The curves remain continuous as expected in the supercritical region, but at the lower pressures they show a strong change of slope close to the WL. In simulations, the WL appears to mark a change in the behaviour of dynamics as well. For the lowest pressures, it is possible to distinguish between a gas-like and a liquid-like behaviour of the diffusion coefficient with the use of the Arrhenius formula where E A is the activation energy. The fits are shown in the inset of the top part of Fig. 3b . For temperatures far from the critical point at the lowest pressures, the diffusion in both the gas-like and in the liquid-like regions is determined by activated processes with different activation energies. The values of E A are reported in the figure caption and they result to be higher in the liquid-like part. For pressures higher than P =250 bar, it becomes more difficult to realize a good fit for the diffusion. From the behaviour of the experimental η and the simulated D , we can extract the points where the curvature changes. To precisely locate the inflection points, we calculated the numerical derivatives of the curves (not shown). We now present the lines calculated at the P- and T -values of the inflection points for both the experimental η and the calculated D , together with the maxima of C P , α P and K T for both experiments and simulations in Fig. 4 . 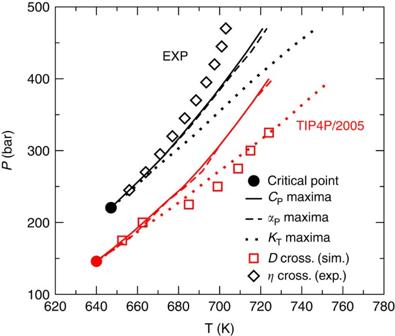Figure 4: Dynamic crossover at the Widom line. The (P,T) location of the viscosity crossovers extracted from experimental data and of diffusion coefficient crossovers extracted from TIP4P/2005 are shown in the figure together with LGCP and thermodynamic response functions maxima from experiments and simulations. Figure 4: Dynamic crossover at the Widom line. The ( P , T ) location of the viscosity crossovers extracted from experimental data and of diffusion coefficient crossovers extracted from TIP4P/2005 are shown in the figure together with LGCP and thermodynamic response functions maxima from experiments and simulations. Full size image It is evident that similar to the thermodynamic response functions, the lines of the dynamic crossovers located through the derivatives of η and D coincide with the WL in approaching the critical point. In particular, the crossover of the experimental viscosity follows the WL for almost 30 K. It is clear from this results that the transport properties of supercritical water are strongly affected by the presence of the WL. We consider the thermodynamic properties of water along the isobars in the supercritical region analysing experimental results and calculations obtained from the TIP4P/2005 model for water. We derive for both experiments and simulations the lines of the maxima of C P , K T and α P in the single-phase region above the critical point. These curves are related to the WL, defined as the line of the maxima of the correlation length. Starting from ( T C and P C ), we find that the curves of the C P , α P and K T maxima coincide in the ( T , P ) plane for a range of circa 30 K and 90 bar, thus following the WL. For higher temperatures and pressures, the C P and α P maxima follow a similar path, while the maxima of K T deviate. Importantly, we test that the WL coincides with a crossover from a liquid-like to a gas-like behaviour witnessed by a crossover in dynamics of viscosity and diffusion coefficient. These results show analogies with the simulation studies of the WL of supercooled water where dynamical changes [11] , [33] , [34] , [35] and structural changes [18] appear on crossing the WL. In particular, for supercooled TIP4P/2005 water it has been shown that the WL corresponds to having equal occurrence of the two local structures, high-density liquid and low-density liquid, involved in the fluctuations [36] . We therefore show that the supercritical state of water can be divided into a gas-like region and a liquid-like region by the WL anticipating the phase separation and the coexistence that is found below the critical point. These results are in line with recent experimental findings on supercritical noble gases [26] , [27] , and together with those indicate a new perspective in the characterization of the fluid–matter thermodynamics of the supercritical state of water and possibly of other liquids with all the important consequences that this can have for many areas of application. The supercritical state cannot, in fact, be considered as an indistinguishable fluid phase any longer. In the future, it would be interesting to extend the study to other water models and to explore with simulations other dynamical and structural features of supercritical water. In noble gases, there is in particular a vivid debate [27] , [37] on whether a dynamical line, called the Frenkel line, can be of use to characterize regions of different dynamical behaviour in the supercritical state. This line is defined as a crossover in positive sound dispersion corresponding to loss of shear stiffness of the liquid and it has been shown to lie, with respect to the WL, in the liquid-like side of supercritical noble gases [37] , [38] . It would be interesting to explore the behaviour of this line in a molecular and network forming liquid, like water. Besides, it would be of great relevance also to extend the present study to other fluids such as CO 2 whose supercritical state is of uttermost importance in green chemistry. Experimental data The data on supercritical water are obtained from the IAPWS-95/IAPS-EoS, based on experimental data. The EoS is provided by the NIST Chemistry WebBook, at the site http://webbook.nist.gov/chemistry/fluid/ . Computer simulation model We performed simulations using the TIP4P/2005 model for water. TIP4P/2005 (ref 28 ) is a re-parametrized version of the ‘classical’ TIP4P model [39] and it is widely employed. In particular, it was shown to be the best rigid and non-polarizable potential for the reproduction of many features of experimental water [29] . Method of simulation Molecular dynamics simulations were performed in a cubic box containing 4,096 water molecules with an initial density ρ =1.0 g cm −3 . For each pressure, we first equilibrate the system at each temperature for 0.1 ns and then execute production runs of 1 ns from T =600 K to T =800 K, with Δ T =5 K. The simulated isobars are for pressures P n =150+25 n bar ( n =1,...,10). As the critical pressure of the TIP4P/2005 model is P c =146 bar, our isobars never cross the liquid–gas first-order phase transition line. The simulations are run in the NPT ensemble, with a time step for the integration of the equation of motion of 1 fs. We control the temperature using the Nosé–Hoover thermostat [40] , [41] and the pressure by the Parrinello–Rahman barostat [42] , [43] . The short-range interactions are cut off at 1 nm. The electrostatics is dealt with by using the Particle Mesh Ewald algorithm. The simulations are run using GROMACS (versions 4.5.3 and 4.5.5) [44] . For the calculation of the diffusion coefficient, the first and the last 10% of the run are excluded from the linear fit of the mean square displacement. How to cite this article: Gallo, P. et al. Widom line and dynamical crossovers as routes to understand supercritical water. Nat. Commun. 5:5806 doi: 10.1038/ncomms6806 (2014).